Structure-based discovery of Middle East respiratory syndrome coronavirus fusion inhibitor A novel human coronavirus, Middle East respiratory syndrome coronavirus (MERS-CoV), has caused outbreaks of a SARS-like illness with high case fatality rate. The reports of its person-to-person transmission through close contacts have raised a global concern about its pandemic potential. Here we characterize the six-helix bundle fusion core structure of MERS-CoV spike protein S2 subunit by X-ray crystallography and biophysical analysis. We find that two peptides, HR1P and HR2P, spanning residues 998–1039 in HR1 and 1251–1286 in HR2 domains, respectively, can form a stable six-helix bundle fusion core structure, suggesting that MERS-CoV enters into the host cell mainly through membrane fusion mechanism. HR2P can effectively inhibit MERS-CoV replication and its spike protein-mediated cell–cell fusion. Introduction of hydrophilic residues into HR2P results in significant improvement of its stability, solubility and antiviral activity. Therefore, the HR2P analogues have good potential to be further developed into effective viral fusion inhibitors for treating MERS-CoV infection. A decade ago, a novel human coronavirus, termed Severe Acute Respiratory Syndrome coronavirus (SARS-CoV), caused a large epidemic with a case fatality rate of ~10%, creating worldwide panic and economic damage [1] , [2] . In 2012, another novel coronavirus, termed Middle East respiratory syndrome coronavirus (MERS-CoV), emerged in the Middle East [3] . MERS-CoV infection results in SARS-like disease with multiorgan failure [4] . As of 11 November 2013, WHO had been informed of 153 confirmed cases, including 64 deaths (a case fatality rate of 42%) [5] . The reports of clusters that have occurred among family contacts or in health-care settings have indicated its person-to-person transmissibility through close contacts, raising concerns over its pandemic potential [3] , [6] , [7] , [8] . Therefore, it is essential to identify the drug targets in the life cycle of MERS-CoV, and in turn, to develop anti-MERS therapeutics to treat patients with MERS-CoV infection and combat any potential pandemic. MERS-CoV is an enveloped positive-sense single-stranded RNA virus with a genome size of ~30 kb (ref. 3 ). It belongs to the lineage C betacoronavirus in the family Coronaviridae within the order Nidovirales . Genetically, it is closer to the bat coronaviruses HKU4 and HKU5 than SARS-CoV [9] , [10] . Nonetheless, its broader animal species and human tissue tropism suggests that it has jumped interspecies barriers to cause human infection, although its origin is still elusive [9] , [11] , [12] . Similar to SARS-CoV, MERS-CoV binds to the host cell through the interaction between the receptor-binding domain in its spike (S) protein S1 subunit [13] , [14] , [15] , [16] , [17] and its receptor dipeptidyl peptidase-4 (DPP4, also known as CD26) [18] . We hypothesized that the S2 subunit of MERS-CoV would then change conformation by inserting its fusion peptide into the target cell membrane, forming a six-bundle (6-HB) fusion core between the heptad repeat 1 and 2 (HR1 and HR2) domains in the S2 subunit, thus bringing the viral and cell membranes into close apposition to facilitate fusion, and, in turn, releasing the viral genetic materials into the cytoplasm [19] , [20] . If this hypothesis is proven, then the HR1 in the 6-HB could serve as a target for developing MERS-CoV fusion inhibitors, like those against HIV infection, such as the peptides SJ-2176 and T20 (enfuvirtide) [21] , [22] , [23] . Here we solve the crystal structure of the 6-HB formed by MERS-CoV S protein HR1 and HR2 domains. Based on the structure, we design several peptides spanning the HR1 and HR2 sequences, respectively. We find that one of the HR2 peptides, HR2P, potently inhibits MERS-CoV infection and its S protein-mediated cell–cell fusion. Introduction of Glu, Lys or Arg residue into HR2P leads to the increase of its stability, solubility and anti-MERS-CoV activity, suggesting that these peptides can be further developed as effective MERS therapeutics. Overall structure of the MERS-CoV fusion core From the NCBI, we obtained the full-length amino-acid sequence of MERS-CoV (hCoV–EMC) S protein (GenBank: JX869059.1) [24] , whose S2 subunit contains, by multiple sequence alignment with SARS-CoV S protein, an N-terminal fusion peptide (FP, residues 943–982), an HR1 domain (residues 984–1,104), an HR2 domain (residues 1,246–1,295), a transmembrane domain (residues 1,296–1,318) and an intracellular domain (residues 1,319–1,353) ( Fig. 1a ). 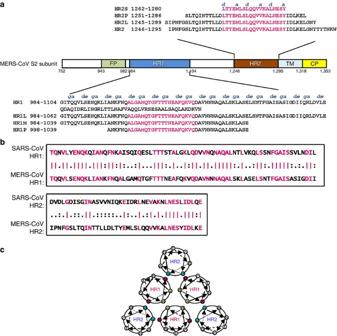Figure 1: Design of peptides and fusion proteins based on the sequence analysis of the MERS-CoV S protein S2 subunit. (a) Schematic representation of MERS-CoV S protein S2 subunit. FP, fusion peptide; HR1, heptad repeat 1 domain; HR2, heptad repeat 2 domain; TM, transmembrane domain; CP, cytoplasmic domain. Residue numbers of each region correspond to their positions in S protein of MERS-CoV. The corresponding sequences of the HR1 and HR2 domains and the designed peptides (HR1L, HR1M, and HR1S, HR2L, HR2M, and HR2S) are shown in the diagram. The fragments in the HR1 and HR2 domains highlighted in magenta are the regions involved in the formation of the 6-HB core of MERS-CoV S protein, according to our X-ray crystal structure. (b) Sequence similarities between the N-terminal portion of HR1 domain (residues 986–1,055) in S2 of MERS-CoV and that of SARS-CoV (residues 894–963) and N-terminal portion of the HR2 domain (residues 1,246–1,285) in S2 of MERS-CoV and that of SARS-CoV (residues 1,144–1,183). Identical amino-acid residues are highlighted in magenta. (c) Formation of 6-HB between HR1 and HR2. The internal trimer is formed through the interaction of the residues located at theaanddpositions (shown in yellow) in three HR1, and 6-HB is formed through the interaction of the residues located at theeandgpositions (shown in magenta) in the HR1 and theaanddpositions (shown in blue) in HR2. Figure 1: Design of peptides and fusion proteins based on the sequence analysis of the MERS-CoV S protein S2 subunit. ( a ) Schematic representation of MERS-CoV S protein S2 subunit. FP, fusion peptide; HR1, heptad repeat 1 domain; HR2, heptad repeat 2 domain; TM, transmembrane domain; CP, cytoplasmic domain. Residue numbers of each region correspond to their positions in S protein of MERS-CoV. The corresponding sequences of the HR1 and HR2 domains and the designed peptides (HR1L, HR1M, and HR1S, HR2L, HR2M, and HR2S) are shown in the diagram. The fragments in the HR1 and HR2 domains highlighted in magenta are the regions involved in the formation of the 6-HB core of MERS-CoV S protein, according to our X-ray crystal structure. ( b ) Sequence similarities between the N-terminal portion of HR1 domain (residues 986–1,055) in S2 of MERS-CoV and that of SARS-CoV (residues 894–963) and N-terminal portion of the HR2 domain (residues 1,246–1,285) in S2 of MERS-CoV and that of SARS-CoV (residues 1,144–1,183). Identical amino-acid residues are highlighted in magenta. ( c ) Formation of 6-HB between HR1 and HR2. The internal trimer is formed through the interaction of the residues located at the a and d positions (shown in yellow) in three HR1, and 6-HB is formed through the interaction of the residues located at the e and g positions (shown in magenta) in the HR1 and the a and d positions (shown in blue) in HR2. Full size image To understand the structural basis of the interactions between HR1 and HR2 regions of MERS-CoV, a fusion protein containing the major parts of HR1 (residues 984–1,062) and HR2 (residues 1,245–1,289) with a short linker (SGGRGG) in between ( Fig. 1a ) was constructed for crystallographic study. Compared with SARS-CoV, these two functional zones possess moderate homology in that the amino acid ratio of HR1 and HR2 is 56.3 and 33%, respectively ( Fig. 1b ). The residues at the a and d positions or e and g positions in the HR1 helix participating in the interaction with another HR1 helix or with HR2 helix, respectively, as well as those at the a and d positions in HR2 helix involving in interaction with HR1 helices ( Fig. 1c ) are labelled above the peptides ( Fig. 1a ). The crystal structure of HR1-L6-HR2 shows a canonical 6-HB structure ( Fig. 2 ). Taking a rod-like shape with a length of ~112 Å and a diameter of ~27 Å, the MERS-CoV S protein fusion core contains a parallel trimeric coiled coil of three HR1 helices (grey in Fig. 2a ) around which three HR2 helices are entwined (green in Fig. 2a ) in an oblique antiparallel manner. The helices constituting the 6-HB are formed by residues 987–1,062 in the HR1 domain and residues 1,263–1,279 in the HR2 domain, respectively. Additionally, residues 1,283–1,285 fold into a one-turn 3 10 helix at the very C-terminal of HR1-L6-HR2 fusion protein. 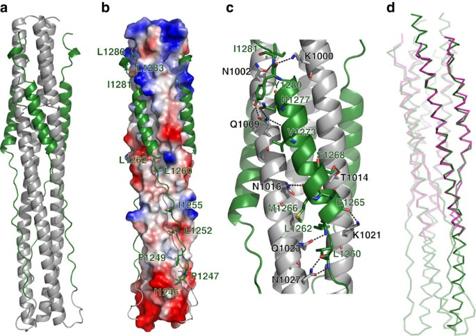Figure 2: Crystal structure of MERS-CoV 6-HB. (a) Cartoon representation of the MERS-CoV fusion core structure, in which the HR1 and HR2 segments are coloured in grey and green, respectively. (b) Electrostatic potential surface of three central HR1 helices, as calculated using PyMOL (DeLano Scientific, Palo Alto, CA, USA), shows the hydrophobic grooves formed between each of two adjacent HR1 helices. Three HR2 segments in the grooves are shown in cartoon representation. (c) The hydrophilic interactions between HR1 and HR2 helices. The residues involved in forming hydrogen bonds are shown in stick representation and are properly labelled, as well as hydrogen bonds in dark grey dashed lines. (d) Superimposition between fusion core structure of MERS-CoV (green) and SARS-CoV (magenta). Figure 2: Crystal structure of MERS-CoV 6-HB. ( a ) Cartoon representation of the MERS-CoV fusion core structure, in which the HR1 and HR2 segments are coloured in grey and green, respectively. ( b ) Electrostatic potential surface of three central HR1 helices, as calculated using PyMOL (DeLano Scientific, Palo Alto, CA, USA), shows the hydrophobic grooves formed between each of two adjacent HR1 helices. Three HR2 segments in the grooves are shown in cartoon representation. ( c ) The hydrophilic interactions between HR1 and HR2 helices. The residues involved in forming hydrogen bonds are shown in stick representation and are properly labelled, as well as hydrogen bonds in dark grey dashed lines. ( d ) Superimposition between fusion core structure of MERS-CoV (green) and SARS-CoV (magenta). Full size image Interactions between MERS-CoV fusion core helices As we predicted, the interaction between one HR2 helix and its two adjacent HR1 helices is predominantly hydrophobic, consistent with the previously determined fusion core structures of other coronaviruses [25] , [26] , [27] , [28] , [29] , [30] , [31] , [32] . Three deep hydrophobic grooves, which are clamped between each two adjacent HR1 helices, become the binding sites of three HR2 helices ( Fig. 2b ). Although a notable difference in length is observed between the HR1 and HR2 helices (~21 turns versus ~4.5 turns), both the N- and C-terminal tails of the HR2 region pack in an orderly manner against the hydrophobic grooves of a central three-helical coiled coil, mainly through hydrophobic interactions involving I1246, P1247, F1249, L1252, I1255, L1260 and L1262 at the N-terminal portion and I1281, L1283 and L1286 at the C-terminal portion of the HR2 helix ( Fig. 2b ). The hydrophilic interactions between one HR2 helix and its two neighbouring HR1 helices consist of 15 hydrogen bonds, mostly distributed in the regions around the N- and C-terminal ends of the HR2 helices ( Fig. 2c ). Around the N-terminal portion of the HR2 helix, its L1260, L1262 and E1265 form four hydrogen bonds with Q1023 and N1027 of its fused HR1 helix and K1021 of the adjacent HR1 helix. Around the C-terminal portion of the HR2 helix, its V1273, N1277, Y1280 and I1281 form hydrogen bonds with N1002 and Q1009 of its fused HR1 helix and K1000 of the adjacent HR1 helix. The relatively concentrated hydrogen bonds constitute two anchoring points at both ends of one short HR2 helix, called N-Cap and C-Cap conformation, which further stabilize its binding with the central hydrophobic grooves. Before this study, the fusion core structures of five coronaviruses, including SARS-CoV, MHV, hCoV-NL63, hCoV-229E and TGEV, had been solved [25] , [26] , [27] , [28] , [29] , [30] , [31] , [32] . Here we further compared the 6-HB core structures of MERS-CoV and SARS-CoV with those of MHV and hCoV-NL63 since the fusion core structures of hCoV-229E and TGEV are not available in PDB. The fusion core of MERS-CoV adopts a similar fold as that of SARS-CoV ( Fig. 2d ), but it is different from those of MHV and hCoV-NL63 ( Fig. 3 ). In the MHV structure, a single-turn α-helix could be observed in the N-terminal region of HR2, which could not be found in MERS-CoV and other coronaviruses. In the hCoV-NL63 structure, the HR2 segment forms regular helices packing against the central HR1 core, especially in the C-terminal region of HR2, which is quite different from the HR2 of MERS-CoV. In contrast, the 6-HB core structure of MERS-CoV S protein could be superimposed on that of SARS-CoV S protein with a root mean square deviation of 0.61 Å for the 63 Cα atoms of three HR1 helices ( Fig. 2d ). Besides the HR2 helices, the N- and C-terminal tail regions of HR2 share similar conformations between MERS-CoV and SARS-CoV, indicating that the tail regions interact with the hydrophobic grooves in a conserved manner in addition to the highly conserved 6-HB. 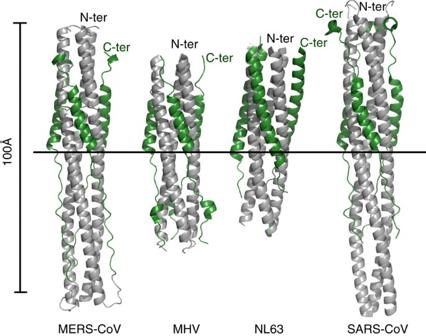Figure 3: Recapitulation of current structural data on the fusion core of coronavirus S2 protein. Coloured identically, the three HR1 segments are in grey, while the HR2 segments in forest green. The very left panel displays the structure of MERS-Cov fusion core in this report. The PDB codes of other structures are 1WDF for MHV, 2IEQ for hCoV-NL63 and 1WYY for SARS. The images are all the same scale, with a horizontal bar to provide the alignment means. The N- and C-terminal ends of the constructs have also been marked. Figure 3: Recapitulation of current structural data on the fusion core of coronavirus S2 protein. Coloured identically, the three HR1 segments are in grey, while the HR2 segments in forest green. The very left panel displays the structure of MERS-Cov fusion core in this report. The PDB codes of other structures are 1WDF for MHV, 2IEQ for hCoV-NL63 and 1WYY for SARS. The images are all the same scale, with a horizontal bar to provide the alignment means. The N- and C-terminal ends of the constructs have also been marked. Full size image Biophysical characterization of the HR1 and HR2 peptides and the 6-HB To further demonstrate the interaction between HR1 and HR2 in the 6-HB, as displayed by the crystal structure, and to determine the stability of the 6-HB, we designed and synthesized two individual peptides, designated HR1P and HR2P, overlapping the regions involving interaction between the HR1 and HR2 domains in the crystal structure ( Fig. 1a ). Since native polyacrylamide-gel electrophoresis (N-PAGE) is under nondenaturing conditions and has been successfully used for testing the formation of 6-HB core structures in other class 1 fusion proteins [20] , [33] , [34] , we used N-PAGE to investigate whether HR1P could interact with HR2P to form 6-HB. Similar to the HR1 peptides from SARS-CoV S protein and HIV-1 gp41 [20] , [33] , [34] , HR1P alone showed no band in the gel (lane 1, Fig. 4a and Supplementary Fig. 9a ) since it carries net positive charges and thus moves up and off the gel under the native electrophoresis condition. HR2P alone exhibited a band at the lower position in the gel (lane 2, Fig. 4a and Supplementary Fig. 9a ), while the mixture of HR1P/HR2P showed a new band at the upper position in the gel (lane 3, Fig. 4a and Supplementary Fig. 9a ), which is expected to be the oligomeric complex formed by HR1P and HR2P. However, we could not judge whether or not this oligomeric complex was a 6-HB since the migration speed of a molecule or a complex in N-PAGE depends on both the net charge and the size. It was reported that the 6-HB complexes formed by HR1 and HR2 of MHV-A59 and SARS-CoV are stable under SDS–PAGE condition without heating the samples at 100 °C before loading [35] . Accordingly, we analysed the HR1P and HR2P peptides, as well as their mixture, using 15% SDS polyacrylamide protein gel (NEXT GEL, Amersco). The result showed that HR1P and HR2P migrated in the gel to a location corresponding to a molecular weight of 3–4 kDa, while the HR1P/HR2P complex migrated to a position corresponding to a molecular mass of ~26 kDa. The theoretical mass of the 6-HB formed by HR1P and HR2P is 25.8 kDa ( Fig. 4b and Supplementary Fig. 9b ). These results therefore suggest that HR1P could interact with HR2P to form a 6-HB. 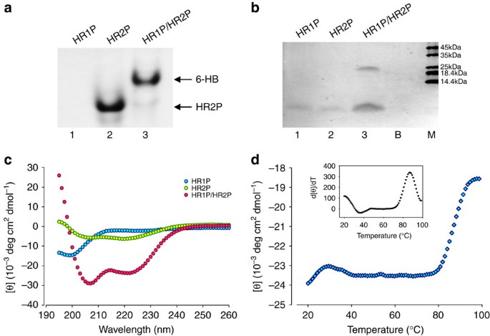Figure 4: Biophysical analysis of the HR1P and HR2P peptides and their complex. (a) Determination of the 6-HB formation between HR1P and HR2P by N-PAGE. The mixture of HR1P and HR2P at the final concentration of 35 μM was incubated at 25 °C for 30 min before being loaded into the gel. (b) Molecular mass determined by gel electrophoresis. Samples of each peptide with 50 μM were incubated, diluted 1:1 (v/v) with 2 × Laemmli sample buffer at room temperature and loaded into the gel. B, blank; M, marker. (c) Secondary structures of HR1P, HR2P and HR1P/HR2P complex in phosphate buffer: CD spectra for HR1P (10 μM), HR2P (10 μM) and their complex in phosphate buffer (pH 7.2) at 4 °C. (d) CD signal at 222 nm for the HR1P/HR2P complex as a function of temperature. Insert: curve of the first derivative (d[θ]/dT) against temperature (T), which was used to determine theTm value. Figure 4: Biophysical analysis of the HR1P and HR2P peptides and their complex. ( a ) Determination of the 6-HB formation between HR1P and HR2P by N-PAGE. The mixture of HR1P and HR2P at the final concentration of 35 μM was incubated at 25 °C for 30 min before being loaded into the gel. ( b ) Molecular mass determined by gel electrophoresis. Samples of each peptide with 50 μM were incubated, diluted 1:1 ( v / v ) with 2 × Laemmli sample buffer at room temperature and loaded into the gel. B, blank; M, marker. ( c ) Secondary structures of HR1P, HR2P and HR1P/HR2P complex in phosphate buffer: CD spectra for HR1P (10 μM), HR2P (10 μM) and their complex in phosphate buffer (pH 7.2) at 4 °C. ( d ) CD signal at 222 nm for the HR1P/HR2P complex as a function of temperature. Insert: curve of the first derivative (d[ θ ]/d T ) against temperature ( T ), which was used to determine the T m value. Full size image Circular-dichroism (CD) spectroscopy was then used to investigate the secondary structures of HR1P and HR2P, as well as the HR1P/HR2P complex, and to determine thermal stability of the HR1P/HR2P complex. As shown in Fig. 4c , the HR1P displayed a random coil structure, whereas HR2P exhibited a relatively low α-helicity in phosphate buffer (pH 7.2). The mixture of HR1P/HR2P at equimolar concentration showed a helical complex, characterized by the saddle-shaped negative peak in the far UV region of the CD spectrum (with minima at 208 and 222 nm) and a remarkable increase of molar ellipticity ([ θ ]) at 222 nm. This helical bundle showed strong thermal stability in phosphate buffer with a T m of ~87 °C ( Fig. 4d ), which is similar to that of the SARS-CoV S HR1-L6-HR2 complex (85 °C) [31] . Together with the crystal structural information, the above results confirmed that the peptides derived from HR1 and HR2 domains of MERS-CoV S protein could be used to form 6-HB, which mimics the fusion core structure in vitro . Therefore, the HR1P/HR2P complex provides a useful model as a basis for studying the detailed structure of the MERS-CoV 6-HB core and designing candidate MERS-CoV fusion inhibitors. Inhibition of MERS-CoV S protein-mediated cell–cell fusion To determine whether the HR1P and HR2P peptides are able to inhibit MERS-CoV fusion with the target cell, we developed an MERS-CoV S protein-mediated cell–cell fusion assay using 293T cells that can instantaneously express MERS-CoV S protein and EGFP (293T/MERS/EGFP) as the effector cells and Huh-7 cells that express DPP4, the receptor of MERS-CoV, as the target cells. The 293T cells expressing EGFP only (293T/EGFP) were included as the control. After 293T/MERS/EGFP cells and Huh-7 cells were co-cultured at 37 °C for 4 h, the number of 293T/MERS/EGFP cells fused with Huh-7 cells was counted, and the percent inhibition of a peptide on MERS-CoV S protein-mediated cell–cell fusion was calculated (see Methods). We found that Huh-7 cells could not fuse with 293T/EGFP cells in the absence of MERS-CoV S protein expression, while they could effectively fuse with 293T/MERS/EGFP cells. The fusion between Huh-7 and 293T/MERS/EGFP cells was significantly blocked by HR2P at 10 μM ( Fig. 5a ). The MERS-CoV S protein-mediated cell–cell fusion at the early stage (4 h) could not be observed under an inverted microscope with visible light ( Fig. 5a ). Forty-eight hours later, many more Huh-7 cells could fuse with 293T/MERS/EGFP cells to form big syncytia, which could be easily observed under both fluorescence and light microscopes ( Fig. 5b ), while no syncytium was shown when Huh-7 cells were co-cultured with 293T/EGFP cells and when HR2P peptide was presented in the Huh-7 and 293T/MERS/EGFP cell co-culture ( Fig. 5b ). 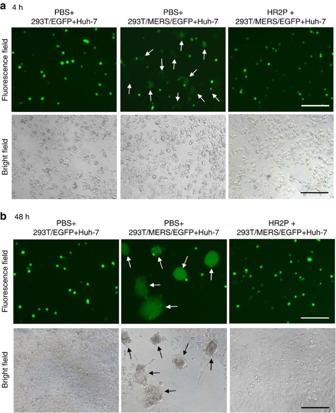Figure 5: Images of MERS-CoV S protein-mediated cell–cell fusion and syncytium formation. (a) MERS-CoV S protein-mediated cell–cell fusion. After Huh-7 cells were co-cultured with 293T/EGFP (left) or 293T/MERS/EGFP cells in the absence (middle) or presence (right) of 10 μM of HR2P at 37 °C for 4 h, cell–cell fusion was photographed under an optical microscope with fluorescence (top) or visible light (bottom). The arrows show the EGFP-labelled cells fused with unlabelled Huh-7 cells (top, middle). (b) MERS-CoV S protein-mediated syncytium formation. After Huh-7 cells were co-cultured with 293T/EGFP (left) or 293T/MERS/EGFP cells in the absence (middle) or presence (right) of 10 μM of HR2P, cell–cell fusion was photographed under an optical microscope with fluorescence or visible light. The arrows show the syncytia formed between 293T/MERS/EGFP and Huh-7 cells (middle). Scale bars, 200 μm. Figure 5: Images of MERS-CoV S protein-mediated cell–cell fusion and syncytium formation. ( a ) MERS-CoV S protein-mediated cell–cell fusion. After Huh-7 cells were co-cultured with 293T/EGFP (left) or 293T/MERS/EGFP cells in the absence (middle) or presence (right) of 10 μM of HR2P at 37 °C for 4 h, cell–cell fusion was photographed under an optical microscope with fluorescence (top) or visible light (bottom). The arrows show the EGFP-labelled cells fused with unlabelled Huh-7 cells (top, middle). ( b ) MERS-CoV S protein-mediated syncytium formation. After Huh-7 cells were co-cultured with 293T/EGFP (left) or 293T/MERS/EGFP cells in the absence (middle) or presence (right) of 10 μM of HR2P, cell–cell fusion was photographed under an optical microscope with fluorescence or visible light. The arrows show the syncytia formed between 293T/MERS/EGFP and Huh-7 cells (middle). Scale bars, 200 μm. Full size image We then compared the inhibitory activity of the peptides HR1P, HR2P, T20 (an anti-HIV-1 peptide) [22] and SC-1 (a peptide derived from the HR2 region of SARS-CoV S protein) [20] on MERS-CoV S-mediated cell–cell fusion. As shown in Fig. 6a , HR1P, T20 and SC-1 exhibited no significant inhibitory activity at the concentration up to 40 μM, while HR2P showed potent inhibitory effect, with IC 50 of ~0.8 μM. These results suggest that HR2P could specifically interact with the viral HR1 domain to form heterologous 6-HB and block viral fusion core formation, resulting in inhibition of MERS-CoV S protein-mediated membrane fusion. 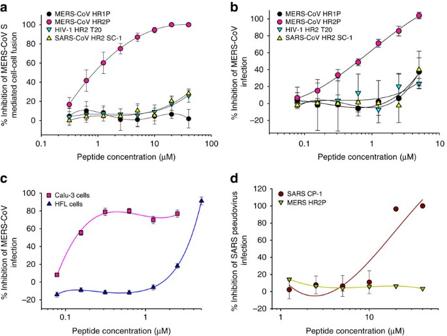Figure 6: Inhibition of peptides derived from the HR1 and HR2 regions in S2 subunit of MERS-CoV S protein on MERS-CoV infection. (a) Inhibitory activity of HP1P and HR2P peptides on MERS-CoV S protein-mediated cell–cell fusion. The HIV-1 HR2-peptide T20 was used as a control. The number of 293T/MERS/EGFP cells fused or unfused with Huh-7 cells were counted under an inverted fluorescence microscope, and the percentage of inhibition was calculated as described in the Methods. (b) Inhibitory activity of HP1P and HR2P peptides on MERS-CoV replication. The HIV-1 HR2-peptide T20 and SARS-CoV HR2 peptide SC-1 were used as controls. (c) Inhibitory activity of HR2P peptide on MERS-CoV replication in Calu-3 and HFL cells. The HIV-1 HR2-peptide T20 and SARS-CoV HR2 peptide SC-1 were used as controls. (d) Inhibitory activity of MERS-CoV HR2 peptide HR2P and SARS-CoV HR2 peptide SC-1 on SARS-CoV infection. The HIV-1 HR2-peptide T20 was used as the control. The cytopathic effect caused by MERS-CoV replication was assessed with MTT assay (bandc), while the SARS-CoV pseudovirus infection in 293T/ACE2 cells was detected by luciferase assay (d). The percentage of inhibition was calculated as described in the Methods. Experiments were performed in triplicate, and the data are expressed as means±s.d. (error bar). The experiment was repeated twice, and similar results were obtained. Figure 6: Inhibition of peptides derived from the HR1 and HR2 regions in S2 subunit of MERS-CoV S protein on MERS-CoV infection. ( a ) Inhibitory activity of HP1P and HR2P peptides on MERS-CoV S protein-mediated cell–cell fusion. The HIV-1 HR2-peptide T20 was used as a control. The number of 293T/MERS/EGFP cells fused or unfused with Huh-7 cells were counted under an inverted fluorescence microscope, and the percentage of inhibition was calculated as described in the Methods. ( b ) Inhibitory activity of HP1P and HR2P peptides on MERS-CoV replication. The HIV-1 HR2-peptide T20 and SARS-CoV HR2 peptide SC-1 were used as controls. ( c ) Inhibitory activity of HR2P peptide on MERS-CoV replication in Calu-3 and HFL cells. The HIV-1 HR2-peptide T20 and SARS-CoV HR2 peptide SC-1 were used as controls. ( d ) Inhibitory activity of MERS-CoV HR2 peptide HR2P and SARS-CoV HR2 peptide SC-1 on SARS-CoV infection. The HIV-1 HR2-peptide T20 was used as the control. The cytopathic effect caused by MERS-CoV replication was assessed with MTT assay ( b and c ), while the SARS-CoV pseudovirus infection in 293T/ACE2 cells was detected by luciferase assay ( d ). The percentage of inhibition was calculated as described in the Methods. Experiments were performed in triplicate, and the data are expressed as means±s.d. (error bar). The experiment was repeated twice, and similar results were obtained. Full size image Inhibition of MERS-CoV replication by HR2P peptide We then tested the potential inhibitory activity of the HR1P and HR2P peptides, with anti-HIV peptide T20 and anti-SARS-CoV peptide SC-1 as controls, on MERS-CoV replication in Vero cells that express DPP4 (ref. 37 ). As shown in Fig. 6b , HR2P could significantly inhibit MERS-CoV replication in Vero cells in a dose-dependent manner, with an IC 50 value of ~0.6 μM, while HR1P, T20 and SC-1 peptides exhibited no significant inhibition at the concentration up to 5 μM. These results suggest that HR2P could specifically inhibit MERS-CoV infection by targeting the HR1 domain in the S2 subunit of the S protein. We further tested the inhibitory activity of HR2P peptide in Calu-3 (human lung adenocarcinoma cell line) and HFL cells (embryonic lung fibroblast cell line). Notably, HR2P could inhibit MERS-CoV infection in Calu-3 cells (IC 50 =0.6 μM) in a manner equal to that observed in Vero cells (IC 50 =0.6 μM), while the same peptide was much less effective in inhibiting MERS-CoV infection in HFL cells (IC 50 =13.9 μM) ( Fig. 6c ), suggesting that MERS-CoV may enter these cells through different pathways, thereby having different sensitivity to the fusion inhibitor HR2P peptide when it enters different target cells. MERS-CoV HR2P could not inhibit SARS-CoV pseudovirus infection in 293T/ACE2 cells at the concentration as high as 20 μM, while the SARS-CoV HR2 peptide SC-1was effective in inhibiting SARS-CoV infection ( Fig. 6d ), indicating that HR2P peptide is a MERS-CoV-specific fusion inhibitor. HR2P inhibits MERS-CoV infection by targeting the viral entry step Using a time-of-addition assay, we found that HR2P lost most of its anti-MERS-CoV activity 4 h after addition of the virus to cells ( Supplementary Fig. 1 ), suggesting that the tested HR2P may target the early stage of virus entry, that is, fusion between the viral envelope and the target cell membranes, which is supported by the evidence that HR2P is highly effective in inhibiting MERS-CoV S protein-mediated cell–cell fusion ( Fig. 6a ) and syncytium formation ( Fig. 5 ). Lack of cytotoxicity of the HR1P and HR2P peptides We then tested the potential cytotoxicity of the HR1P and HR2P peptides on the 293T, Huh-7 and Vero cells that were used for the viral inhibition assays in this study ( Supplementary Fig. 2 ). Neither peptide had significant cytotoxicity to these cells at the concentration up to 1,000 μM. The selectivity index (SI=CC 50 /IC 50 ) of HR2P is >1,667, suggesting that HR2P is an effective MERS-CoV fusion inhibitor with low or no in vitro toxic effect. Optimization of peptides derived from HR1 and HR2 domains MERS-CoV S protein contains a long HR1 sequence, but a shorter HR2 sequence ( Figs 1 and 2 ). The HR1P peptide contains 42 amino acids, a length similar to HR2P. HR1P lacks anti-MERS-CoV activity ( Fig. 6 ), possibly because it is too short. Therefore, we synthesized a medium long peptide, HR1M (56-mer: residues 984–1,039), and expressed a long peptide, HR1L (79-mer: residues 984–1,062). We also synthesized a longer HR2 peptide, HR2L (45-mer: residues 1,245–1,289) and a shorter HR2 peptide HR2S (19-mer: residues 1,262–1,280) ( Fig. 1a ). By comparing the secondary structures of these individual peptides, we found that the 79-mer HR1L peptide formed α-helical structure with 34.5% helicity, while neither the 56-mer HR1M nor the 42-mer HR1P could form α-helical structure ( Supplementary Fig. 3a ). Interestingly, the 36-mer HR2P peptide was in α-helical conformation with 18.5% helicity, while both the 45-mer HR2L peptide and the 19-mer HR2S peptide exhibited random structure in PBS ( Supplementary Fig. 3b ). The α-helicity of the HR1L/HR2P complex (84.3%) and HR1M/HR2P complex (79.9%) was slightly higher than that of HR1P/HR2P complex (71.8%), while the α-helicity of the HR1L/HR2L complex and HR1L/HR2P complex was significantly higher than that of the HR1L/HR2S complex (34.3%). Notably, the T m values of the HR1L/HR2L complex (>99 °C), HR1L/HR2P complex (>99 °C) and HR1M/HR2P complex (98 °C) were higher than that of HR1P/HR2P complex (87 °C), while the T m values of the above complexes were significantly higher than that of the HR1L/HR2S complex (57.5 °C) ( Table 1 ), confirming that the longer peptides generally form more stable fusion core than the shorter peptides [38] , [39] . These results suggest that both HR2L and HR2P peptides are long enough to form 6-HB coiled coil structure with all three HR1 peptides, while HR1S peptide is too short to form the typical fusion core structure with HR1 peptides. Table 1 The α -helicity and T m value of complexes formed by the HR1 and HR2 peptides. Full size table We then compared the inhibitory activity of the longer and shorter HR2 peptide on MERS-CoV S-mediated cell–cell fusion with that of HR2P peptide. While the 19-mer short HR2 peptide, HR2S showed no anti-MERS-CoV activity, the inhibitory activity of the 45-mer long HR2 peptide, HR2L (IC 50 : 0.5 μM) showed marginal improvement over that of the 36-mer HR2P peptide (IC 50 : 0.8 μM). Like HR1P, peptides HR1L and HR1M exhibited no inhibitory activity on MERS-CoV S-mediated cell–cell fusion ( Supplementary Fig. 4 ). Improvement of HR2P peptide by introducing charged residues To increase the stability, solubility and antiviral activity of the HIV-1 gp41 HR1 peptide C34, it was mutated by introducing Glu (E) and Lys (K) residues at the i to i +4 or i to i +3 arrangements. Using a similar approach, we introduced two point mutations into HR2P-M1 peptide, including T1263E ( e ) and L1267R ( b) , and 7 point mutations into HR2P-M2 peptide, including T1263E ( e ), L1267K ( b ), S1268K ( c ), Q1270E ( e ), Q1271E ( f ), A1275K ( c ) and N1277E ( e ). Based on the crystal structure of MERS-CoV fusion core ( Fig. 2 ), none of these mutations was expected to block interaction between HR1 and HR2, since the mutated residues were not located at the a and d positions in the helical wheel of HR2 ( Fig. 1c ). It was expected that these mutations would lead to formation of E–K, K–E or E–R salt-bridge at the i to i+ 4 arrangements, such as 1263E–1267K in HR2P-M1, and 1263E–1267K and 1271E–1275K in HR2P-M2, as well as formation of E–K, K–E or E–R salt-bridge at i to i +3 arrangements, such as 1265E–1268K and 1274K–1277E in HR2P-M2. Other introduced E or K mutations were expected to increase hydrophilicity, thus enhancing the water solubility. In both mutants, as expected, the α-helicity of HR2P-M1 (36.4%) and HR2P-M2 (42.4%) was significantly higher than that of HR2P (18.2%). The α-helicity and T m values of HR1P/HR2P-M1 and HR1P/HR2P-M2 complexes were also higher than that of HR1P/HR2P complex ( Table 2 ), confirming that the introduction of salt-bridges could increase the stability of the helical peptide. The solubility of HR2P-M1 and HR2P-M2 in H 2 O was increased by ~68-fold and 1,786-fold, respectively, while their inhibitory activity on MERS-CoV S-mediated cell–cell fusion was increased by ~9 and 69%, respectively ( Table 2 ). These results are consistent with those obtained by Otaka et al . [40] , suggesting that their approach is also very useful for designing HR2 peptides with improved stability, solubility and anti-MERS-CoV activity. Table 2 The biophysical properties and biological activity of HR2P mutants. Full size table The recent outbreaks of a SARS-like disease with a high fatality rate caused by the novel coronavirus MERS-CoV has raised global concerns over its pandemic potential [3] , [4] , calling for further understanding of its fusion and entry mechanisms in order to develop MERS-CoV fusion/entry inhibitors as therapeutics for treatment of MERS-CoV infection. Based on our previous experience in research on HIV-1 and SARS-CoV fusion inhibitors [20] , [21] , we studied the structure and function of the HR1 and HR2 domains in the S protein S2 subunit of MERS-CoV, particularly the 6-HB fusion core formed by the HR1 and HR2 domains, in order to elucidate the viral fusion mechanism with the aim of designing novel candidate MERS-CoV fusion inhibitors. By constructing the fusion protein HR1-L6-HR2, we successfully generated a crystal and solved the canonical 6-HB structure ( Fig. 2 ). Based on the crystal structure, we found that the regions spanning residues 998–1,039 and 1,251–1,286 in the HR1 and HR2 domains, respectively, mainly participate in the HR1 and HR2 interaction, in a manner similar to the HR1 and HR2 domains in S proteins of SARS-CoV and other coronaviruses ( Fig. 3 ). We then synthesized the two peptides, HR1P and HR2P, characterizing them and their complex by biophysical experiments. We noticed that the peptides could form 6-HB with strong thermal stability, confirming that HR1P and HR2P could interact with each other to form a stable 6-HB core structure. Based on the fusion model of HIV-1 and SARS-CoV, in addition to the results obtained from this study, we proposed a model of plasma membrane fusion that elucidates the fusogenic mechanism mediated by MERS-CoV S protein ( Supplementary Fig. 5 ). In the early 1990s, Jiang et al . [21] and Wild et al . [22] discovered that synthetic peptides derived from the HR2 domain of HIV-1 were highly potent HIV fusion inhibitors. One of the HR2 peptides, T20 (brand name: Fuzeon; generic name: enfuvirtide), was licensed by the US FDA in 2003 for the treatment of HIV infection [41] . In 2004, we found that a peptide (CP-1) derived from the HR2 domain of SARS-CoV S protein exhibited moderate anti-SARS-CoV activity (IC 50 =19 μM) [20] . Xu et al . [26] and Tripet et al . [35] solved the crystal structure of the 6-HB formed by the HR1 and HR2 peptides derived from the SARS-CoV S protein, but they did not show whether or not their HR2 peptides had antiviral activity. Here we tested the potential inhibitory activity of the HR1P and HR2P peptides on MERS-CoV S protein-mediated cell–cell fusion and MERS-CoV replication. We found that HR2P peptide was potent in inhibiting MERS-CoV S protein-mediated cell–cell fusion and syncytium formation. HR2P could also effectively inhibit MERS-CoV replication in Vero cells with an IC 50 of ~0.6 μM, which is ~31-fold more potent than the HR2 peptide SC-1 against SARS-CoV replication in Vero E6 cells [20] . In general, the antiviral activity of HR2 peptides from an enveloped virus with class I membrane fusion protein can be correlated with their length, that is, peptides with longer sequences tend to exhibit better antiviral activity [42] . In the present study, we found that the HR2S peptide with 19 amino acids exhibited no anti-MERS-CoV activity, while the HR2L peptide with 45 amino acids showed marginally improved inhibitory activity over that of the 36-mer HR2P peptide. However, since it is much more difficult and expensive to synthesize a 45-mer peptide than a 36-mer peptide, we select the HR2P peptide for further development. Like the HR1 peptides derived from Env of other enveloped viruses with class I fusion proteins [23] , [38] , [43] , [44] , none of the MERS-CoV HR1 peptides exhibited anti-MERS-CoV activity, possibly because isolated HR1 peptides cannot automatically form an active HR1 trimer and have a tendency to aggregate in physiological solution [38] , [44] in the absence of HR2 peptide from the exposure of the hydrophobic interface ( Fig. 1c ). However, an HR1 peptide may become active if it forms a trimer after it is conjugated with a trimerization motif, such as foldon. We previously demonstrated that N28, an HR1 peptide derived from the HIV-1 gp41, lacked anti-HIV-1 activity, whereas N28Fd, in which a foldon motif is added to the C terminus of N28, possessed highly potent anti-HIV-1 activity [45] . One may question why the peptide derived from the HR2 domain of MERS-CoV S protein is more effective in inhibiting MERS-CoV infection than the HR2 peptide SC-1 in protecting against SARS-CoV infection. One of the explanations is that like HIV-1, MERS-CoV enters the host cell primarily through plasma membrane fusion, while SARS-CoV gets into its target cells perhaps mainly via endosomal membrane fusion. Chan et al . [37] have observed that syncytial formation is very prominent in MERS-CoV-infected cell cultures, while it was not found in SARS-CoV-infected cell cultures. In this study, the co-culture of 293T cells expressing MERS-CoV S protein and Huh-7 cells carrying DPP4 exhibited significant cell–cell fusion and syncytial formation ( Fig. 5 ). Chan et al . [37] have also shown that human lung adenocarcinoma cell line, Calu-3 and embryonic lung fibroblast cell line HFL are highly susceptible to MERS-CoV infection. Interestingly, however, MERS-CoV-infected Calu-3 can form significant syncytia, whereas MERS-CoV-infected HFL cells cannot, suggesting that MERS-CoV may enter these cells through different pathways. In the present study, we tested the inhibitory activity of HR2P peptide in Calu-3 and HFL cells and found that HR2P could inhibit MERS-CoV infection in Calu-3 cells just as effectively as Vero cells, while HR2P was about 22-fold less effective in inhibiting MERS-CoV infection in HFL cells. These findings suggest that MERS-CoV enters into Calu-3 and Vero cells mainly through the plasma membrane fusion route, and, as a result, it is particularly sensitive to inhibition by MERS-CoV fusion inhibitor HR2P, while the virus might enter HFL cells mainly via endocytosis route and, hence, would be relatively resistant to blockade by HR2P peptide. Gierer et al . [46] showed that the MERS-CoV S protein was activated by TMPRSS2 (type II transmembrane serine proteases) and endosomal cathepsins, while Shirato et al . [47] demonstrated that simultaneous treatment with TMPRSS2 and cathepsin L inhibitors completely blocked virus entry into Vero-TMPRSS2 cells, indicating that MERS-CoV employs both the cell surface and the endosomal pathway to infect Vero-TMPRSS2 cells. After uptake of the virus into endosomes, MERS-CoV S protein is activated by pH-dependent cysteine protease Cathepsin L. Therefore, cathepsin L inhibitor is expected to stop lysosomal entry of the virus after uptake by endocytosis. While TMPRSS2 activates the S protein close to the cell surface, its inhibitor may stop the uptake by direct fusion between viral and cytoplasmic membranes. Since the cell–cell fusion depends on the direct membrane fusion without preceding endocytoisis and endosomal uptake, it is expected that cathepsin L inhibitors will not interfere with the cell–cell fusion, but TMPRSS2 inhibitors may do it. Therefore, it will be interesting to determine whether cell type-specific differences in susceptibility to inhibition by the fusion inhibitors correlate with differences in susceptibility to inhibition by cathepsin L and TMPRSS2 inhibitors as well as HR1-targeted fusion inhibitors. By comparing the 6-HB core structures of the MERS-CoV and SARS-CoV S proteins, we noted that obvious differences of some critical residues in their protein sequences might influence the detailed interactions. First, the residues Q1020/D1024 in HR1 domain of MERS-CoV S2 are able to form hydrogen bond, which may increase the stability of the HR1-trimer [48] . However, the corresponding residues G928/D932 in the HR1 domain of SARS-CoV S2 subunit (PDB ID: 1WYY) are incapable of forming this strong interaction ( Supplementary Fig. 6 ) [28] . Second, the binding between D1261 and T1263 and between E1278 and K1274 in HR2 domain of MERS-CoV S2 subunit is stronger than that between Q1161 and N1159 and between E1276 and K1172 in the HR2 domain of SARS-CoV S2 subunit, respectively ( Supplementary Fig. 7 ), suggesting that these two hydrogen bonds in MERS-CoV S2 subunit provide force to stabilize the HR2 helix conformation [49] . Third, there is a hydrogen bond between Q1009 in HR1 and Y1280 in HR2 in MERS-CoV S2, while the corresponding residues Q917 in HR1 and L1178 in HR2 in the SARS-CoV S2 are unable to form the intermolecular hydrogen bond ( Supplementary Fig. 8 ). All these findings suggest that the association between the viral HR1 and HR2 domains in MERS-CoV S2 may be stronger than that found in SARS-CoV S2. Consequently, the HR2 peptide of MERS-CoV S2 may have higher binding affinity and hence higher antiviral activity than the corresponding HR2 peptide of SARS-CoV S2 subunit. Based on the crystal structure of the 6-HB of MERS-CoV S2, HR2P peptide could be modified in order to improve its stability, solubility and antiviral activity using a similar approach described by Otaka et al . [40] by introducing EK mutations, including those forming intramolecular salt-bridges. We thus designed and synthesized two HR2P mutants, HR2P-M1 and HR2P-M2, with 2 and 7 mutations, respectively, some of which could form intramolecular salt-bridges at the i to i+ 4 or at the i to i+ 3 arrangements ( Fig. 2 ). Indeed, both HR2P-M1 and HR2P-M2 and their complexes with HR1P peptide are more stable than HR2P peptide. The water-solubility of HR2P-M1 and HR2P-M2 is ~68-fold and 1,786-fold higher than the HR2P peptide, respectively. Their anti-MERS-CoV activity is moderately improved ( Table 2 ). These results are consistent with those obtained by Otaka et al . [40] , who found that the anti-HIV-1 HR2 peptide C34 with EK mutation (SC34EK) displayed significantly improved stability and water solubility, and moderately improved anti-HIV-1 activity, compared with the wild-type C34 peptide, confirming that this approach can also be used to improve stability, solubility and antiviral activity of HR2 peptides derived from MERS-CoV S protein. Nevertheless, other approaches, such as replacement of the natural amino acids in an HR2 peptide with nonnatural amino acids (for example, D-amino acids) or addition of cholesterol or fatty acid to an HR2 peptide [50] , [51] may also be used to extend the half-life of the MERS-CoV HR2 peptide. Considering the current absence of specific anti-MERS-CoV drug [52] , analogues of HR2P with improved anti-MERS-CoV activity could be developed on a fast-track as a viral entry inhibitor-based anti-MERS-CoV drug for clinical use to treat patients with MERS-CoV infection, much like the anti-HIV peptide T20 (enfuvirtide) for the treatment of HIV infection [41] . However, unlike T20 that has to be used for many months or years in treating HIV infection, it is only necessary to administer the MERS-CoV entry inhibitors for a short period at the early stage of the MERS-CoV infection to ameliorate the infection and save lives. Cells The cell lines 293T, Vero E6 and Calu-3 were obtained from ATCC (Manassas, VA, USA). Huh-7 cell line was from Cell Bank of Chinese Academy of Science (Shanghai, China). The above cell lines were cultured in Dulbecco’s Modified Eagle Medium (DMEM) supplemented with 10% fetal bovine serum (FBS). Expression and purification of fusion protein HR1-L6-HR2 To express the fusion protein HR1-L6-HR2, the nucleotide sequence encoding the MERS-CoV HR2 region (residues 1,245–1,289) was attached to the 3′ end of the HR1 region (residues 984–1,062) with a short linker (L6: SGGRGG) in between by overlapping PCR as previously described for constructing SARS-CoV (or HIV-1) 6-HB (ref. 25 ). The whole sequence was subcloned into the pET-28a vector with an artificial SUMO-tag. The pET-28a-SUMO-HR1-L6-HR2-transformed E. coli cells were induced with 1 mM IPTG, incubated overnight at 16 °C and purified by Ni-NTA affinity resin (Qiagen, Valencia, CA, USA). His-SUMO-tag was cleaved off with Ulp1 enzyme at 4 °C for 2 h. The purified HR1-L6-HR2 was applied onto a Superdex-75 gel filtration column (GE Healthcare, Piscataway, NJ, USA). Fractions containing HR1-L6-HR2 trimer were collected and concentrated by ultrafiltration [53] . Crystallization and structure determination The fusion protein HR1-L6-HR2 was crystallized at 16 °C using the hanging drop, vapor-diffusion method. The crystals were grown on a siliconized cover clip by equilibrating a mixture containing 1 μl protein solution (20 mg ml −1 HR1-L6-HR2 trimer in 20 mM Tris–HCl (pH 8.0), 150 mM NaCl) and 1 μl reservoir solution (0·1 M HEPES:NaOH (pH 7.5), 25% ( w / v ) PEG3350) against 400 μl reservoir solution. After 1 week, single crystals formed and were flash-frozen by liquid nitrogen for future data collection. On the in-house (Institute of Biophysics, Chinese Academy of Sciences) X-ray source (MicroMax 007 generator (Rigaku, Japan) combined with Varimax HR optics (Rigaku, Japan)), HR1-L6-HR2 crystals at 100 K were diffracted to 2.3-Å resolution at a wavelength of 1.5418 Å. A native set of X-ray diffraction data was collected with R-AXIS IV++ detector (Rigaku, Japan) with an exposure time of 2 min per image and was indexed and processed using HKL2000 (ref. 54 ). The space group of the collected data set is P321. Molecular replacement was performed with PHENIX.phaser to solve the phasing problem, using the SARS-CoV S protein core structure (PDB code 1WYY) as a search model [28] . The final model was manually adjusted in COOT and refined with PHENIX.refine [55] , [56] . Data collection statistics and refinement statistics are given in Table 3 . Coordinates were deposited in the RCSB Protein Data Bank (PDB code: 4NJL). Table 3 Data collection and refinement statistics. Full size table Biophysical analysis of HR1P and HR2P peptides The MERS-CoV peptides, including HR1P (residues 998–1,039), HR1M (residues 984–1,039), HR1L (residues 984–1,062), HR2L (residues 1,245–1,289), HR2P (residues 1,251–1,286) and a shorter HR2 peptide HR2S (19-mer: residues 1,262–1,280) ( Fig. 1a ); the SARS-CoV peptides SC-1 (residues 1,152–1,188) and the HIV-1 gp41 peptide T20 (residues 638–673) were all synthesized with standard solid-phase methods [57] . The peptides were found to be ~95% pure by high performance liquid chromatography (HPLC) and identified by laser desorption mass spectrometry (PerSeptive Biosystems, Framingham, MA, USA). The secondary structure of the peptides was determined by CD spectroscopy as previously described [33] , [44] , [58] . The individual peptides or peptide mixtures were diluted in phosphate buffer (50 mM sodium phosphate, pH 7.2) at the final concentration of 10 μM, and the CD spectra were acquired on a J-815 spectropolarimeter (Jasco, Inc. Japan). The CD data were presented as mean residue ellipticity and the [ θ ] 222 value of −33,000 deg cm 2 dmol −1 was taken to correspond to 100% α-helical content [23] , [58] . Thermal denaturation was monitored at 222 nm by application of a thermal gradient of 5 °C min −1 . The melting curve was smoothed, and the midpoint of the thermal unfolding transition ( T m) values was calculated with Jasco software utilities. Native N-PAGE was conducted as previously described [20] . Equimolar mixtures of HR1P and HR2P peptides (35 μM in phosphate buffer, pH 7.2) were incubated at 25 °C for 30 min. After the addition of Tris-glycine native sample buffer (TIANDZ, Inc., China), the mixture was loaded on the 18% Tris-glycine gel with a Tricine glycine running buffer (pH 8.3). Gel electrophoresis was carried out with constant 125 V at room temperature for 2 h and then stained with Coomassie blue. The images were visualized by the FluorChem Imaging System (Alpha Innotech/ProteinSimple, Santa Clara, CA, USA). Sodium dodecyl sulphate polyacrylamide gel electrophoresis (SDS–PAGE) was performed to measure the molecular mass of the peptides and their complex [35] . The individual peptide HR1P or HR2P, or their equimolar mixture (50 μM of each peptide), dissolved in PBS was incubated at room temperature. Samples were then diluted with 1 volume of 2 × Laemmli sample buffer [35] and loaded onto the 15% NEXT GEL (Amresco, Solon, OH, USA), which was run at 150 V for 60 min at room temperature until the tracking dye reached the bottom edge of the gel. The gel was then stained with Coomassie blue. Inhibition of MERS-CoV S protein-mediated cell–cell fusion MERS-CoV S protein-mediated cell–cell fusion was assessed using a method similar to that for determining HIV-1 Env-mediated cell–cell fusion [59] . Briefly, 293T cells were transfected with the plasmid pAAV-IRES-EGFP encoding the EGFP (293T/EGFP) or pAAV-IRES-MERS-EGFP encoding the MERS-CoV S protein and EGFP (293T/MERS/EGFP) and cultured in DMEM containing 10% FBS at 37 °C for 48 h. Huh-7 cells (5 × 10 4 ) expressing the MERS-CoV receptor DPP4 were incubated in 96-well plates at 37 °C for 5 h, followed by the addition of 1 × 10 4 293T/EGFP or 293T/MERS/EGFP cells, respectively, in the absence or presence of the test peptides at graded indicated concentrations. After co-culture at 37 °C for 4 h, the 293T/MERS/EGFP cells (293T/EGFP cells were used as the negative control) fused or unfused with Huh-7 cells were counted under an inverted fluorescence microscope (Nikon Eclipse Ti-S). The fused cell was much larger by at least twofold than the unfused cell, and the intensity of fluorescence in the fused cell was weaker than that of the unfused cell as a result of the diffusion of EGFP from one cell to two or more cells (see Fig. 5a ). The percent inhibition of cell–cell fusion was calculated using the following formula: (1−( E − N )/( P − N )) × 100. ‘ E ’ represents the % cell–cell fusion in the experimental group. ‘ P ’ represents the % cell–cell fusion in the positive control group, to which no inhibitor was added. ‘ N ’ is the % cell–cell fusion in negative control group, in which 293T/MERS/EGFP cells were replaced by 293T/EGFP cells. The concentration for 50% inhibition (IC 50 ) was calculated using the CalcuSyn software kindly provided by Dr T.C. Chou [60] . After further co-culture at 37 °C for 48 h, syncytium formation between 293T/MERS/EGFP and Huh-7 could be observed under an inverted microscope with or without fluorescence ( Fig. 5b ), and the syncytia were photographed for the record. Inhibition of MERS-CoV replication The inhibitory activity of the synthetic peptides on MERS-CoV replication in Vero cells was tested using a previously described method with some modifications [37] . Briefly, 20 TCID 50 (50% tissue-culture infectious dose) of MERS-CoV was mixed with an equal volume of a peptide at graded concentrations and incubated at 37 °C for 30 min. Then, the mixture was inoculated in triplicate wells of 96-well microtiter plates with preformed monolayers of Vero cells. After incubation at 37 °C for 2 h, the supernatants were removed and fresh medium was added. On day 3 after infection, the cytopathic effect caused by MERS-CoV replication was assessed by MTT assay, and the IC 50 value was calculated by using the CalcuSyn software [60] . Inhibition of pseudotyped SARS-CoV and MERS-CoV infection SARS or MERS pseudovirus bearing SARS-CoV or MERS-CoV S protein, respectively, and a defective HIV-1 genome that expresses luciferase as reporter was prepared by co-transfecting 293T cells with the plasmid pNL4-3.luc.RE (encoding Env-defective, luciferase-expressing HIV-1) and pcDNA3.1-MERS-CoV-S plasmid [61] , [62] . To detect the inhibitory activity of a peptide on infection by SARS or MERS pseudovirus, ACE2-transfected 293T (293T/ACE2) cells and Huh-7 cells (10 4 per well in 96-well plates) were respectively infected with SARS or MERS-CoV pseudovirus, in the presence or absence of a peptide at indicated concentration. The culture was re-fed with fresh medium 12 h post-infection and incubated for an additional 72 h. Cells were washed with PBS and lysed using lysis reagent included in a luciferase kit (Promega). Aliquots of cell lysates were transferred to 96-well Costar flat-bottom luminometer plates (Corning Costar), followed by the addition of luciferase substrate (Promega). Relative light units were determined immediately in the Ultra 384 luminometer (Tecan US) [63] . Cytotoxicity assay The cytotoxicity of the peptides to the cells (293T, Huh-7 cells and Vero E6 cells) that were used for testing cell fusion and MERS-CoV replication was detected by using a Cell Counting Kit (CCK-8, Dojindo, Kumamoto, Japan) following the manufacturer’s instruction. Briefly, 100 μl cells (1 × 10 5 ml −1 ) were seeded into the wells of a 96-well microtiter plate and incubated at 37 °C for 12 h. Then, 5 μl of a peptide at graded concentrations was added. After incubation at 37 °C for 2 days, 10 μl of CCK-8 solution were added, followed by an additional incubation for 2 h. The absorbance was measured at 450 nm. Accession code: Structure coordinates have been deposited in the RCSB Protein Data Bank under accession code 4NJL . How to cite this article: Lu, L. et al . Structure-based discovery of Middle East respiratory syndrome coronavirus fusion inhibitor. Nat. Commun. 5:3067 doi: 10.1038/ncomms4067 (2014).